Mast cells form antibody-dependent degranulatory synapse for dedicated secretion and defence Mast cells are tissue-resident immune cells that play a key role in inflammation and allergy. Here we show that interaction of mast cells with antibody-targeted cells induces the polarized exocytosis of their granules resulting in a sustained exposure of effector enzymes, such as tryptase and chymase, at the cell–cell contact site. This previously unidentified mast cell effector mechanism, which we name the antibody-dependent degranulatory synapse (ADDS), is triggered by both IgE- and IgG-targeted cells. ADDSs take place within an area of cortical actin cytoskeleton clearance in the absence of microtubule organizing centre and Golgi apparatus repositioning towards the stimulating cell. Remarkably, IgG-mediated degranulatory synapses also occur upon contact with opsonized Toxoplasma gondii tachyzoites resulting in tryptase-dependent parasite death. Our results broaden current views of mast cell degranulation by revealing that human mast cells form degranulatory synapses with antibody-targeted cells and pathogens for dedicated secretion and defence. Mast cells are tissue-resident immune cells particularly enriched in regions such as skin, gastrointestinal tract and airways that are exposed to the external environment. The functions of mast cells in immunity are manifold. Beyond their well-established key role in allergy [1] , mast cells can sense danger signals [2] , elicit inflammatory responses [3] , participate in pathogen elimination [4] and regulate T-cell-mediated immune responses [5] , [6] . Mast cells are characterized by a cytoplasm filled with secretory granules containing a large array of preformed mediators [7] . The matrix of these granules is composed of proteoglycans, mostly constituted of heparin and its core peptide serglycin, a highly anionic macromolecular complex in which mast cell bioactive mediators are embedded [8] , [9] . During the degranulation process, granule membranes fuse with each other and with the plasma membrane leading to the release of granule content into the surrounding environment. Some mediators, such as histamine, serotonin or β-hexosaminidase, quickly diffuse from the released granules, whereas others, such as tryptase, chymase or tumour-necrosis factor (TNF), dissociate more slowly allowing granule remnants to keep their biological activity for a prolonged time [8] , [10] , [11] , [12] . Granule enzymes play numerous roles in immune responses [13] , [14] . Notably, human tryptase can favour the recruitment of inflammatory cells by activating endothelial cells via protease-activated receptors such as PAR-2 (refs 15 , 16 , 17 ). Moreover, in vivo studies provided evidence of direct or indirect protective roles of mast cell chymase against infection [18] or vasoactive agents [19] , [20] . Mast cell degranulation is efficiently triggered by Fc receptor aggregation and is followed by a delayed phase of neosynthetized cytokines secretion [7] , [21] , [22] . Human mast cells (hMCs) express constitutively two activating FcR: the high-affinity IgE receptor (FcεRI) and the low-affinity IgG receptor (FcγRIIA) [23] , [24] , [25] . Unlike FcεRI, FcγRIIA cannot bind to monomeric antibodies in the absence of antigen but it can bind to antibodies as multivalent immune complexes with high avidity. Those receptors belong to the immunoreceptor tyrosine-based activation motif (ITAM)-containing superfamily of immunoreceptors and are coupled to a signalling cascade involving src-kinases triggering, [Ca 2+ ] i increase and actin cytoskeleton remodelling [26] , [27] , [28] . Mast cell degranulation is classically studied using soluble stimuli such as secretagogues or antigen/antibody-mediated FcR crosslinking. However, naturally occurring ligands for FcR can also be displayed on the surface of other cells or be immobilized within the extracellular matrix network, thus providing localized stimulation. Studies using supported lipid bilayers showed that localized FcεRI stimulation leads to receptor clustering and signalling and to granule exocytosis [29] , [30] , [31] , [32] . Although surrogate stimulatory surfaces are instrumental to study the dynamics of receptors and associated signalling components, they do not mimic the complex molecular interactions occurring at the cell–cell contact site. Moreover, whether and how IgG-targeted cellular antigens efficiently trigger hMCs during antibody-mediated immune response against pathogens remain to be elucidated. In the present study, we sought to monitor the spatiotemporal dynamics of mast cell degranulation following local stimulation by mean of IgG- or IgE-targeted cell surface antigens. Our results show that FcR triggering by either IgE- or IgG-targeted cell-bound antigens results in a vectorial exposure of granules at the cell–cell contact site that overlies the signalling area. We name this phenomenon antibody-dependent degranulatory synapse (ADDS). Degranulatory synapse is characterized by actin cytoskeleton clearance and allows close contact of the targeted cells with granule bioactive material. ADDS also occurs at the contact site with IgG-opsonized Toxoplasma gondii , resulting in parasite death and in the release of pro-inflammatory cytokines and chemokines. Our work provides a conceptual advance in the field of mast cell biology by widening the current view of mast cell degranulation, classically seen as a response triggered by the aggregation of high-affinity IgE receptors by soluble ligands. Mast cell surface expression of degranulated material Primary hMCs used in this study were derived from CD34 + peripheral blood progenitors [33] . After 8–10 weeks of culture, more than 95% of the generated cells stained metachromatically with acidic toluidine blue and co-expressed CD117, FcεRI and FcγRIIA on their surface and intracellular tryptase and chymase ( Supplementary Fig. 1 ). To define the spatiotemporal characteristics of mast cell degranulation, we set-up a method to monitor, in live cells, the early steps of granule exocytosis using fluorochrome-labelled avidin, a probe that specifically binds heparin contained in mast cell granules [34] . During the degranulation process, granule matrix is externalized and immediately bound by the probe. In a first approach, IgE-sensitized hMCs were stimulated with anti-IgE monoclonal antibody (2.5 μg ml −1 ) in the presence of avidin-sulforhodamine (Av.SRho) and inspected by time-lapse confocal microscopy. As shown in Supplementary Movie 1 and Fig. 1a , this stimulation induced granule budding on the hMC surface as detected by labelling with Av.SRho. Interestingly, although part of the exocyted granules were released in the culture medium, a substantial part of granule content was retained on the hMC surface ( Supplementary Movie 1 ). Measurement of the intensity of the Av.SRho staining using the Region Measurement function of the MetaMorph software showed that degranulation was detectable ~10 min after anti-IgE addition and reached a plateau ~15 min later ( Fig. 1b ). A similar degranulation pattern was obtained when hMCs were triggered by a weak stimulus (0.06 μg ml −1 anti-IgE, Supplementary Fig. 2 and Supplementary Movie 2 ), indicating that the observed phenomenon does not depend on the stimulus strength. We also employed an Annexin-V-binding assay to monitor hMC degranulation following anti-IgE stimulation [35] . The results obtained using this method corroborated the results observed using avidin ( Supplementary Fig. 3 and Supplementary Movie 3 ). Moreover, a similar time-kinetics of degranulation was observed by monitoring β-hexosaminidase release under the same conditions used for time-lapse microscopy ( Supplementary Fig. 4 ). 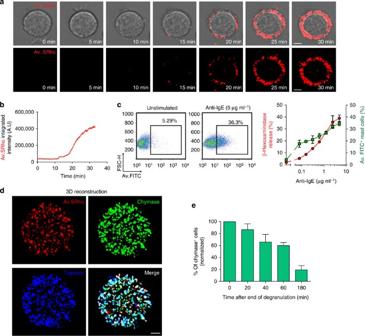Figure 1: Granule-stored bioactive material is displayed on the mast cell surface following degranulation. (a) IgE-sensitized hMCs were stimulated with anti-IgE monoclonal antibody (mAb) in Tyrode’s buffer containing avidin-sulforhodamine (Av.SRho). The stimulus was added at the time 0 of time-lapse recording. Panels show a sequence of snapshots from 1 representative movie out of 15 (seeSupplementary Movie 1). The progressive formation of a corona of degranulated material is depicted. Scale bars, 5 μm. (b) Measurement of mast cell Av.SRho integrated fluorescence intensity (IFI) using the region measurement function of Metamorph Software (data are fromSupplementary Movie 1). (c) Mast cells were stimulated for 30 min with increasing concentrations of anti-IgE mAb. Degranulation was monitored by FACS analysis using Avidin-FITC to stain membrane-bound exocyted granules or by β-hexosaminidase release assay. Representative dot plots of Avidin-FITC staining are shown, numbers indicate the percentage of positive cells. Results (mean±s.e.m.) are from three independent experiments. (d) Mast cells were stimulated as inafor 30 min and settled onto poly-L-lysine-coated slides, fixed and stained for chymase (green) and tryptase (blue). Panels show 3D reconstruction of a z-stack of confocal images. Data are from one representative cell out of ten from three independent experiments. Scale bars, 3 μm. (e) Mast cells were stimulated as inafor 20 min then chilled at 4 °C to stop degranulation. Cells were rested in culture medium at 37 °C for different times and then analysed by flow cytometry for chymase expression. The percentage of chymase+cells after 20 min of stimulation (time 0) was normalized to 100%. It corresponds to 37±3% chymase-positive cells. Data are from three independent experiments. Figure 1: Granule-stored bioactive material is displayed on the mast cell surface following degranulation. ( a ) IgE-sensitized hMCs were stimulated with anti-IgE monoclonal antibody (mAb) in Tyrode’s buffer containing avidin-sulforhodamine (Av.SRho). The stimulus was added at the time 0 of time-lapse recording. Panels show a sequence of snapshots from 1 representative movie out of 15 (see Supplementary Movie 1 ). The progressive formation of a corona of degranulated material is depicted. Scale bars, 5 μm. ( b ) Measurement of mast cell Av.SRho integrated fluorescence intensity (IFI) using the region measurement function of Metamorph Software (data are from Supplementary Movie 1 ). ( c ) Mast cells were stimulated for 30 min with increasing concentrations of anti-IgE mAb. Degranulation was monitored by FACS analysis using Avidin-FITC to stain membrane-bound exocyted granules or by β-hexosaminidase release assay. Representative dot plots of Avidin-FITC staining are shown, numbers indicate the percentage of positive cells. Results (mean±s.e.m.) are from three independent experiments. ( d ) Mast cells were stimulated as in a for 30 min and settled onto poly- L -lysine-coated slides, fixed and stained for chymase (green) and tryptase (blue). Panels show 3D reconstruction of a z-stack of confocal images. Data are from one representative cell out of ten from three independent experiments. Scale bars, 3 μm. ( e ) Mast cells were stimulated as in a for 20 min then chilled at 4 °C to stop degranulation. Cells were rested in culture medium at 37 °C for different times and then analysed by flow cytometry for chymase expression. The percentage of chymase + cells after 20 min of stimulation (time 0) was normalized to 100%. It corresponds to 37±3% chymase-positive cells. Data are from three independent experiments. Full size image We next used avidin-fluorescein isothiocyanate (FITC) staining and fluorescence-activated cell sorting (FACS) analysis to measure the membrane-bound fraction following degranulation for 30 min with different concentrations of anti-IgE. This analysis showed that the per cent of avidin + degranulated cells increased with the strength of stimulation. Interestingly, this readout exhibited sensitivity comparable or even greater than that of the commonly used β-hexosaminidase release measurements ( Fig. 1c ). To test whether key granule-stored effector molecules might be retained on the hMC surface together with the membrane-bound granule matrix, we stained hMCs with antibodies directed against tryptase and chymase 30 min after stimulation. This analysis showed that these two effector molecules were retained on the surface of degranulated hMCs ( Fig. 1d ). To investigate whether hMCs display on their surface bioactive material for a sustained time after degranulation, we measured by FACS analysis the surface exposure of chymase, a molecule that has been reported to remain associated to granule heparin following degranulation [10] . As shown in Fig. 1e , chymase exposure on mast cell surface was sustained for at least 1 h after degranulation, indicating that bioactive material is displayed on degranulated mast cell surface for a prolonged time. These results show that fluorochrome-labelled avidin staining is a useful tool to monitor early degranulation events in mast cells by time-lapse microscopy and FACS analysis. They also show that exocyted granules containing bioactive material can be either released in the medium or stored on the cell surface to display key hMC enzymes for a prolonged time. Polarized degranulation induced by cell-bound ligands The observation that hMCs retain a substantial portion of exocyted material on their surface prompted us to investigate whether they might expose granule content in a vectorial manner when triggered by focused stimuli. To address this point, we used the well-known humanized monoclonal antibody anti-human CD20 (rituximab) to target CD20 that is expressed on B-cell surface. We initially employed a rituximab-based IgE generated by recombinant DNA technology to sensitize hMCs. hMCs were co-cultured in the presence of Av.SRho with CD20 + Epstein–Barr virus-transformed B cells and hMC degranulation was monitored by time-lapse confocal laser-scanning microscopy. Remarkably, as shown in Fig. 2a and Supplementary Movies 4 and 5 , granule release occurred mostly at the contact site between hMCs and B cells. This polarized release was detectable ~10 min after conjugate formation as shown by measurement of the intensity of Av.SRho staining at the cell–cell contact site ( Fig. 2b ). Similar results were obtained when an Annexin-V-binding assays was used to monitor mast cell degranulation ( Supplementary Fig. 5 and Supplementary Movies 6 and 7 ). 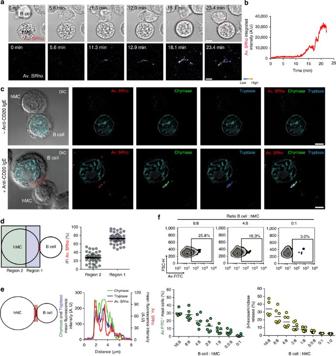Figure 2: Localized FcεRI aggregation by cell-bound ligands initiates polarized mast cell degranulation. (a) Anti-CD20 IgE-sensitized hMCs were incubated with CD20+B cells in Tyrode’s buffer plus Av.SRho. Live cells were imaged for 25 min using a LSM 710 confocal microscope (seeSupplementary Movies 4 and 5). Panels show a sequence of snapshots depicting the interaction between hMC and B cell. Upper panels show differential interference contrast (DIC) plus Av.SRho fluorescence (red); lower panels show the enrichment of Av.SRho signal at the contact site area (pseudocolour scale intensity). Results are from one representative experiment out of five. Scale bars, 5 μm. (b) Av.SRho integrated fluorescence intensity (IFI) measurement at the hMC/B-cell contact site using the Region Measurement Function of MetaMorph software (data are fromSupplementary Movies 4). (c) B cells were incubated for 30 min with hMCs sensitized or not with anti-CD20 IgE, cells were fixed and stained for chymase (green) and tryptase (blue). Individual stainings for a representative conjugate are shown. Scale bars, 5 μm. (d) Quantification of Av.SRho fluorescence in sensitized hMC/B-cell conjugates (n=37, 4 independents experiments) using the Region Measurement function of MetaMorph. Region 1 corresponds to the synaptic area as depicted in the scheme. Av.SRho fluorescence is expressed as percentage of IFI measured in each region. (e) Analysis of chymase, tryptase and Av.SRho fluorescence signal localization using the Linescan function of MetaMorph software. Line scans were calculated using the three red lines shown in the scheme and in the above cell image. The mean of the measured fluorescence intensity along the three indicated lines is plotted against distance. (f) Anti-CD20 IgE-sensitized hMC were co-cultured for 1 h with B cells at different ratio. Supernatants were collected for β-hexosaminidase release assays and cells were stained with Av.FITC and analysed by flow cytometry. Representative dot plots are shown. Numbers indicate the percentage of positive cells. Each dot represents an independent experiment. Figure 2: Localized FcεRI aggregation by cell-bound ligands initiates polarized mast cell degranulation. ( a ) Anti-CD20 IgE-sensitized hMCs were incubated with CD20 + B cells in Tyrode’s buffer plus Av.SRho. Live cells were imaged for 25 min using a LSM 710 confocal microscope (see Supplementary Movies 4 and 5 ). Panels show a sequence of snapshots depicting the interaction between hMC and B cell. Upper panels show differential interference contrast (DIC) plus Av.SRho fluorescence (red); lower panels show the enrichment of Av.SRho signal at the contact site area (pseudocolour scale intensity). Results are from one representative experiment out of five. Scale bars, 5 μm. ( b ) Av.SRho integrated fluorescence intensity (IFI) measurement at the hMC/B-cell contact site using the Region Measurement Function of MetaMorph software (data are from Supplementary Movies 4 ). ( c ) B cells were incubated for 30 min with hMCs sensitized or not with anti-CD20 IgE, cells were fixed and stained for chymase (green) and tryptase (blue). Individual stainings for a representative conjugate are shown. Scale bars, 5 μm. ( d ) Quantification of Av.SRho fluorescence in sensitized hMC/B-cell conjugates ( n =37, 4 independents experiments) using the Region Measurement function of MetaMorph. Region 1 corresponds to the synaptic area as depicted in the scheme. Av.SRho fluorescence is expressed as percentage of IFI measured in each region. ( e ) Analysis of chymase, tryptase and Av.SRho fluorescence signal localization using the Linescan function of MetaMorph software. Line scans were calculated using the three red lines shown in the scheme and in the above cell image. The mean of the measured fluorescence intensity along the three indicated lines is plotted against distance. ( f ) Anti-CD20 IgE-sensitized hMC were co-cultured for 1 h with B cells at different ratio. Supernatants were collected for β-hexosaminidase release assays and cells were stained with Av.FITC and analysed by flow cytometry. Representative dot plots are shown. Numbers indicate the percentage of positive cells. Each dot represents an independent experiment. Full size image Scoring of a significant number of individual conjugates showed that in IgE-sensitized hMC/B-cell conjugates >80% Av.SRho fluorescence was detected at the contact area ( Fig. 2c,d ). We also analysed mast cell/B-cell conjugates in three dimension to assess whole-cell degranulation. This analysis confirmed that granule exocytosis mostly occurred at the cell–cell contact site ( Supplementary Fig. 6 ). Staining with antibodies directed against tryptase and chymase showed that these granule-associated effector molecules co-localized with Av.SRho staining at the cell–cell contact site ( Fig. 2e ). Polarized degranulation was dependent on FcεRI crosslink as it was not observed at the hMC/B-cell contact site in the absence of anti-CD20 IgE sensitization ( Fig. 2c ). We employed both FACS analysis and β-hexosaminidase release assays to evaluate whether hMC stimulation by cell-bound antigens would result in a substantial degranulation. Both assays showed that the extent of degranulation was proportional to the number of stimulating B cells and that at high B-cell/hMC ratios, the amount of β-hexosaminidase released was similar to that induced by optimal concentrations of soluble anti-IgE, indicating that local hMC stimulation induces a substantial response (compared Figs 1c with 2f ). The above results indicate that localized stimulation of mast cells by cell-bound ligands triggers substantial and polarized degranulation. Molecular dynamics at the degranulatory synapse Having observed that hMCs can degranulate in a synaptic mode, we sought to define the molecular mechanisms of localized degranulation. We initially focused on early signalling occurring at the cell–cell contact site in hMCs sensitized with anti-CD20 IgE and interacting with CD20 + B cells. Staining for the FcεRI showed an enrichment of this receptor at the hMC/B-cell contact site ( Fig. 3a ) in the proximity of exocyted Av.SRho + granules. Staining with anti-phosphotyrosines (pTyr) antibodies showed an increased pTyr staining at the hMC/B-cell contact site, beneath the secreted Av.SRho + granules ( Fig. 3c ). Linker for activation of T cells (LAT) phosporylation was also detected at the degranulatory area ( Fig. 3e ). Quantification of morphological data showed that FcεRI, pTyr and phospho-LAT (pLAT) were significantly enriched at the contact area ( Fig. 3b,d,f ). We named the area of polarized degranulation where mast cells cluster ITAM-containing receptors and associated signalling components, ADDS. This area is indeed reminiscent of the T- and B-cell immunological synapses [36] , [37] . 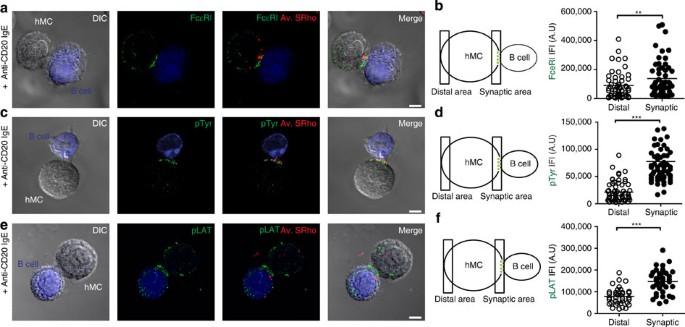Figure 3: FcεRI and phospho-LAT are enriched at the degranulatory synapse. Anti-CD20 IgE-sensitized hMCs were incubated with DDAO-labelled CD20+B cells in Tyrode’s buffer plus Av.SRho for 10 min at 37 °C. Cells were fixed, permeabilized, stained with anti-FcεRI (a,b), anti-pTyr monoclonal antibody (c,d) and anti-phospho-LAT (e,f) and analysed by confocal microscopy. Individual stainings for representative conjugates are shown. Results are from one representative experiment out of three. (b,dandf) quantification of integrated fluorescence intensity (IFI) at the distal and synaptic areas (see schemes) of FcεRI (b;n=56 conjugates), pTyr (d;n=63 conjugates) and pLAT (f;n=36 conjugates) staining. Pairedt-test **P<0.01; ***P<0.001. Scale bars, 5 μm. Figure 3: FcεRI and phospho-LAT are enriched at the degranulatory synapse. Anti-CD20 IgE-sensitized hMCs were incubated with DDAO-labelled CD20 + B cells in Tyrode’s buffer plus Av.SRho for 10 min at 37 °C. Cells were fixed, permeabilized, stained with anti-FcεRI ( a , b ), anti-pTyr monoclonal antibody ( c , d ) and anti-phospho-LAT ( e , f ) and analysed by confocal microscopy. Individual stainings for representative conjugates are shown. Results are from one representative experiment out of three. ( b , d and f ) quantification of integrated fluorescence intensity (IFI) at the distal and synaptic areas (see schemes) of FcεRI ( b ; n =56 conjugates), pTyr ( d ; n =63 conjugates) and pLAT ( f ; n =36 conjugates) staining. Paired t -test ** P <0.01; *** P <0.001. Scale bars, 5 μm. Full size image To gain further insights on the molecular mechanisms of focal mast cell degranulation, we investigated whether remodelling of actin and tubulin cytoskeleton might occur in mast cells upon contact with cognate B cells. As shown in Fig. 4a,b , the area of granule release was characterized by clearance of cortical actin. Conversely, neither microtubule organizing centre (MTOC) nor Golgi apparatus were detected at the cell–cell contact sites, indicating that in hMCs, the polarized release of granules does not require MTOC re-polarization ( Fig. 4c–f ). Enrichment of FcεRI and signalling components and actin clearance were not detected in conjugates formed by nonsensitized hMC and B cells ( Supplementary Fig. 7 ). 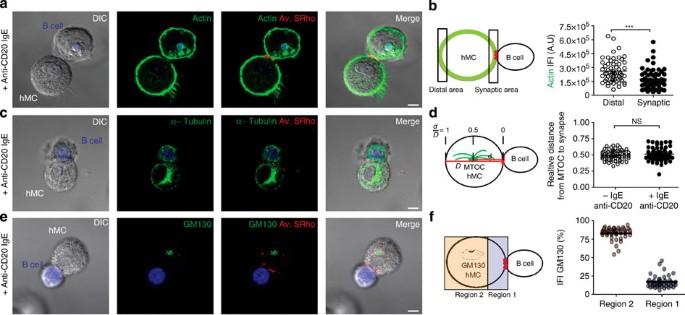Figure 4: F-actin clearance occurs underneath the degranulation area. Anti-CD20 IgE-sensitized hMCs were incubated with DDAO-labelled CD20+B cells in Tyrode’s buffer plus Av.SRho for 30 min at 37 °C. Cells were fixed, permeabilized, stained with phalloidin (a,b), α-tubulin (c,d) and anti-GM130 (e,f) and analysed by confocal microscopy. Representative conjugates are shown. Results are from one representative experiment out of three. (b) Quantification of phalloidin integrated fluorescence intensity (IFI) at the distal and synaptic areas (see scheme;n=59 conjugates) staining. Pairedt-test, ***P<0.001. (d) Measurement of distance of MTOC from the synapse. Plots show the distance from MTOC to the synapse divided by the hMC diameter (d/D) for each conjugate (see scheme). Experiments were performed using either nonsensitized hMC (− anti-CD20 IgE,n=62 seeSupplementary Fig. 7efor a typical image) or sensitized hMC (+ anti-CD20 IgE,n=64). Unpairedt-test, not significant (NS):P>0.05. (f) Quantification of GM130 fluorescence in conjugates (n=45) using the Region Measurement function of MetaMorph. Region 1 corresponds to the synaptic area as depicted in the scheme. GM130 fluorescence is expressed as percentage of IFI measured in each region. Scale bars, 5 μm. Figure 4: F-actin clearance occurs underneath the degranulation area. Anti-CD20 IgE-sensitized hMCs were incubated with DDAO-labelled CD20 + B cells in Tyrode’s buffer plus Av.SRho for 30 min at 37 °C. Cells were fixed, permeabilized, stained with phalloidin ( a , b ), α-tubulin ( c , d ) and anti-GM130 ( e , f ) and analysed by confocal microscopy. Representative conjugates are shown. Results are from one representative experiment out of three. ( b ) Quantification of phalloidin integrated fluorescence intensity (IFI) at the distal and synaptic areas (see scheme; n =59 conjugates) staining. Paired t -test, *** P <0.001. ( d ) Measurement of distance of MTOC from the synapse. Plots show the distance from MTOC to the synapse divided by the hMC diameter ( d / D ) for each conjugate (see scheme). Experiments were performed using either nonsensitized hMC (− anti-CD20 IgE, n =62 see Supplementary Fig. 7e for a typical image) or sensitized hMC (+ anti-CD20 IgE, n =64). Unpaired t -test, not significant (NS): P >0.05. ( f ) Quantification of GM130 fluorescence in conjugates ( n =45) using the Region Measurement function of MetaMorph. Region 1 corresponds to the synaptic area as depicted in the scheme. GM130 fluorescence is expressed as percentage of IFI measured in each region. Scale bars, 5 μm. Full size image Together, the above results reveal that mast cells stimulated by cell-bound antigens form degranulatory synapses that are characterized by localized signalling and actin clearance. Degranulatory synapses are triggered by FcγRIIA engagement As IgG-mediated responses are more frequent than IgE responses and target a larger array of pathogens and as hMCs are known to express additional activating Fc receptors beside the FcεRI (such as FcγRIIA and FcγRI), we investigated whether mast cells might be triggered by IgG-opsonized cells. As shown in Supplementary Movie 8 and Fig. 5a , a Rituximab-opsonized B-cell triggered polarized secretion by hMCs within ~15 min after cell contact. FACS analysis showed that hMCs did not express FcγRI nor FcγRIII in basal conditions while they expressed FcγRIIA ( Fig. 5b ). We thus analysed FcγRIIA localization in hMC/B-cell conjugates by confocal microscopy. As shown in Fig. 5d , an enrichment of FcγRIIA was observed at the synaptic area in parallel with the localized exposure of secreted granules. FcγRIIA staining appeared to be punctate suggesting the presence of receptor clusters at the synapse. Scoring of a significant number of individual hMC/rituximab-opsonized B-cell conjugates confirmed that a large fraction of exocyted material was detected at the synaptic area ( Fig. 5e ) and that FcγRIIA receptors were significantly enriched within this area ( Fig. 5f ). 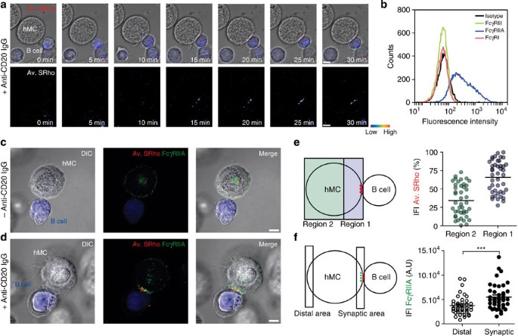Figure 5: Mast cells form degranulatory synapses upon interaction with rituximab-opsonized B cells. B cells were opsonized or not with 1 μg ml−1of anti-CD20 humanized-IgG1 (Rituximab) and loaded with DDAO. Mast cells and B cells were co-cultured in the presence of Av.SRho and monitored by time-lapse microscopy. (a) Sequence of snapshots showing the interaction between hMC and B cells. Live cells were imaged for 30 min using a LSM 710 confocal microscope. Upper panels show DIC plus Av.SRho (red) and DDAO (blue); lower panels show Av.SRho staining in a pseudocolour scale. Data are fromSupplementary Movie 8. Results are from one representative experiment out of five. Scale bars, 5 μm. (b) FACS analysis of FcγRI, FcγRIIA, FcγRIII expression on hMC surface. (c,d) B cells were opsonized (d) or not (c) with rituximab then co-cultured with hMCs for 30 min in the presence of Av.SRho. The cells were fixed and stained for FcγRIIA. The panels show a representative hMC/B-cell conjugate. Scale bars, 5 μm. (e) Quantification of Av.SRho staining in hMC/opsonized B-cell conjugates using the Region Measurement function of MetaMorph. Region 1 corresponds to the synaptic area as depicted in the scheme. Results are expressed as percentage of integrated fluorescence intensity (IFI) measured in each region. (f) Quantification of FcγRIIA IFI at the distal and synaptic areas (see scheme). Fluorescence is expressed as IFI measured in each region. Results are from three independent experiments. Pairedt-test, ***P<0.001. Figure 5: Mast cells form degranulatory synapses upon interaction with rituximab-opsonized B cells. B cells were opsonized or not with 1 μg ml −1 of anti-CD20 humanized-IgG1 (Rituximab) and loaded with DDAO. Mast cells and B cells were co-cultured in the presence of Av.SRho and monitored by time-lapse microscopy. ( a ) Sequence of snapshots showing the interaction between hMC and B cells. Live cells were imaged for 30 min using a LSM 710 confocal microscope. Upper panels show DIC plus Av.SRho (red) and DDAO (blue); lower panels show Av.SRho staining in a pseudocolour scale. Data are from Supplementary Movie 8 . Results are from one representative experiment out of five. Scale bars, 5 μm. ( b ) FACS analysis of FcγRI, FcγRIIA, FcγRIII expression on hMC surface. ( c , d ) B cells were opsonized ( d ) or not ( c ) with rituximab then co-cultured with hMCs for 30 min in the presence of Av.SRho. The cells were fixed and stained for FcγRIIA. The panels show a representative hMC/B-cell conjugate. Scale bars, 5 μm. ( e ) Quantification of Av.SRho staining in hMC/opsonized B-cell conjugates using the Region Measurement function of MetaMorph. Region 1 corresponds to the synaptic area as depicted in the scheme. Results are expressed as percentage of integrated fluorescence intensity (IFI) measured in each region. ( f ) Quantification of FcγRIIA IFI at the distal and synaptic areas (see scheme). Fluorescence is expressed as IFI measured in each region. Results are from three independent experiments. Paired t -test, *** P <0.001. Full size image Taken together with the above results, these data show that crosslinking of IgE or IgG FcRs by cell-bound antigens results in a polarized and sustained exposure of granule content at the mast cell/stimulatory cell contact site. ADDS at the mast cell/ T. gondii contact site We next investigated whether hMCs could form degranulatory synapses upon contact with IgG-opsonized pathogens. As mast cells were previously shown to be recruited and activated at the site of T. gondii infection in rodents [38] , we focused on T. gondii , a widespread parasite known to actively invade any type of nucleated cell, including human white blood cells [39] . T. gondii RH tachyzoites were opsonized with IgG directed against the surface antigen SAG-1 and co-cultured with hMCs. Time-lapse microscopy showed that hMCs exhibited a polarized degranulation towards the invading parasite ( Supplementary Movie 9 and Fig. 6a ). Conversely, when non-opsonized T. gondii were used, they rapidly infected mast cells, without triggering any detectable degranulation process ( Supplementary Movie 10 ). Scoring of hMCs in contact with T. gondii showed that most Av.A488 fluorescence was detected at the site of contact with the parasite ( Fig. 6b,c ). 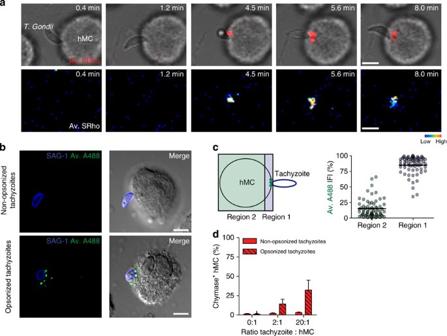Figure 6: OpsonizedT. Gondiitachyzoites induce the formation of degranulatory synapses. (a) Anti-SAG-1 IgG-opsonized tachyzoites were incubated with hMCs in Tyrode’s buffer plus Av.SRho. Live cells were imaged for 25 min using a LSM 710 confocal microscope (seeSupplementary Movie 9). Panels show a sequence of snapshots depicting the interaction between hMC andT. gondii. Upper panels show DIC plus Av.SRho (red); lower panels show Av.SRho staining in a pseudocolour scale. Results are from one representative experiment out of five. Scale bars, 5 μm. (b,c) Tachyzoites opsonized or not with anti-SAG-1 IgG were incubated with hMCs in Tyrode’s buffer plus Av.A488 for 1 h. Cells were fixed and stained for SAG-1 (blue) and analysed by confocal microscopy. (b) Individual stainings for representative conjugates are shown. Scale bars, 5 μm. (c) Quantification of Av.A488 staining in opsonized tachyzoite/hMC conjugates (n=67, from three independent experiments) using the Region Measurement function of MetaMorph. Region 1 corresponds to the synaptic area as depicted in the scheme. Av.A488 fluorescence is expressed as percentage of integrated fluorescence intensity measured in each region. (d) Tachyzoites opsonized or not with anti-SAG-1 IgG were incubated with hMCs (MOI=2 or 20) in Tyrode’s buffer for 4 h. Cells were stained for chymase and analysed by flow cytometry. Results (mean±s.e.m.) are from four independent experiments. Figure 6: Opsonized T. Gondii tachyzoites induce the formation of degranulatory synapses. ( a ) Anti-SAG-1 IgG-opsonized tachyzoites were incubated with hMCs in Tyrode’s buffer plus Av.SRho. Live cells were imaged for 25 min using a LSM 710 confocal microscope (see Supplementary Movie 9 ). Panels show a sequence of snapshots depicting the interaction between hMC and T. gondii . Upper panels show DIC plus Av.SRho (red); lower panels show Av.SRho staining in a pseudocolour scale. Results are from one representative experiment out of five. Scale bars, 5 μm. ( b , c ) Tachyzoites opsonized or not with anti-SAG-1 IgG were incubated with hMCs in Tyrode’s buffer plus Av.A488 for 1 h. Cells were fixed and stained for SAG-1 (blue) and analysed by confocal microscopy. ( b ) Individual stainings for representative conjugates are shown. Scale bars, 5 μm. ( c ) Quantification of Av.A488 staining in opsonized tachyzoite/hMC conjugates ( n =67, from three independent experiments) using the Region Measurement function of MetaMorph. Region 1 corresponds to the synaptic area as depicted in the scheme. Av.A488 fluorescence is expressed as percentage of integrated fluorescence intensity measured in each region. ( d ) Tachyzoites opsonized or not with anti-SAG-1 IgG were incubated with hMCs (MOI=2 or 20) in Tyrode’s buffer for 4 h. Cells were stained for chymase and analysed by flow cytometry. Results (mean±s.e.m.) are from four independent experiments. Full size image The capacity of opsonized T. gondii to trigger degranulation was confirmed by FACS analysis showing that increasing the multiplicity of infection (MOI) of opsonized parasite resulted in the exposure of chymase on an increasing fraction of hMCs ( Fig. 6d ). The comparison of hMC interaction with opsonized versus non-opsonized parasites (shown in Supplementary Movies 9 and 10 ) suggests that hMC degranulation might affect parasite invasion as opsonized T. gondii penetration into degranulating hMCs appeared to be blocked. However, invasion ability of the tachyzoites may also be impaired by SAG-1 antibody coating. To distinguish between the impact of opsonization and degranulation on the detected defective parasite function, we took advantage of the fact that only a fraction of the cultured hMC population degranulated upon FcR triggering using either opsonized T. gondii ( Supplementary Fig. 8 ) or anti-IgE monoclonal antibodies ( Fig. 1c ). We could therefore specifically evaluate the impact of degranulation on opsonized T. gondii . We investigated the viability of opsonized T. gondii in contact with hMCs having or not degranulated after 4 h of co-culture by using a viability probe compatible with fixation procedures. This analysis showed that more than 70% of parasites that had triggered polarized degranulation by hMCs were dead, whereas only 20% of parasites contacting non-degranulated mast cells were dead ( Fig. 7a,b ). 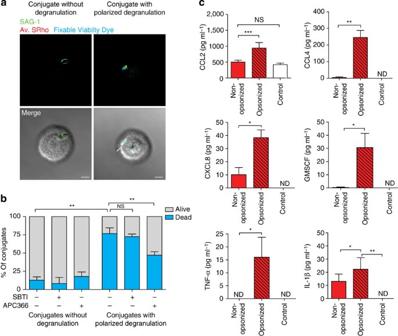Figure 7: Degranulatory synapse formation correlates with parasite death and is accompanied by mast cell activation to cytokine and chemokine production. (a) Anti-SAG-1 IgG-opsonized tachyzoite were incubated with hMCs (MOI=2) in Tyrode’s buffer for 4 h. Cells were incubated for 30 min at 4 °C with avidin-SRho (red), Fixable Viability Dye (cyan) and goat anti-mouse IgG2a-A488 (to stain SAG-1, green) then fixed and analysed by confocal microscopy. Representative conjugates from non-degranulated hMCs (left panels) and degranulated hMCs (right panels) are shown. Scale bars, 5 μm. (b) Frequency of live or dead (Fixable Viability Dye+) tachyzoites among the two groups (mean±s.e.m.) with or without chymase (SBTI) or tryptase (APC 366) inhibitors. At least 80 conjugates were randomly selected for each experimental condition. Data are from three independent experiments. Pairedt-test, **P<0.01. (c) hMCs and tachyzoites (opsonized or not, MOI=2) were co-cultured in Tyrode’s buffer for 6 h; supernatants were harvested and analysed for indicated cytokines. Results (mean±s.e.m.) are from six independent experiments. Wilcoxon pairedt-test, not significant (NS):P>0.05; *P<0.05; **P<0.01; ***P<0.001; ND, not detected. Figure 7: Degranulatory synapse formation correlates with parasite death and is accompanied by mast cell activation to cytokine and chemokine production. ( a ) Anti-SAG-1 IgG-opsonized tachyzoite were incubated with hMCs (MOI=2) in Tyrode’s buffer for 4 h. Cells were incubated for 30 min at 4 °C with avidin-SRho (red), Fixable Viability Dye (cyan) and goat anti-mouse IgG2a-A488 (to stain SAG-1, green) then fixed and analysed by confocal microscopy. Representative conjugates from non-degranulated hMCs (left panels) and degranulated hMCs (right panels) are shown. Scale bars, 5 μm. ( b ) Frequency of live or dead (Fixable Viability Dye + ) tachyzoites among the two groups (mean±s.e.m.) with or without chymase (SBTI) or tryptase (APC 366) inhibitors. At least 80 conjugates were randomly selected for each experimental condition. Data are from three independent experiments. Paired t -test, ** P <0.01. ( c ) hMCs and tachyzoites (opsonized or not, MOI=2) were co-cultured in Tyrode’s buffer for 6 h; supernatants were harvested and analysed for indicated cytokines. Results (mean±s.e.m.) are from six independent experiments. Wilcoxon paired t -test, not significant (NS): P >0.05; * P <0.05; ** P <0.01; *** P <0.001; ND, not detected. Full size image As mast cell tryptase and chymase stay associated with granule matrix on the mast cell surface following degranulation ( Fig. 1d,e ), we investigated T. gondii mortality in the presence of specific tryptase (APC 366) or chymase (soybean tryptase inhibitor, SBTI) inhibitors. Treatment with the chymase inhibitor SBTI did not affect parasite mortality. Conversely, treatment with the tryptase inhibitor APC 366 induced a significant decrease in the number of dead parasites found in contact with degranulated mast cells, indicating that this enzyme plays an important role in parasite death. Treatment with APC 366 inhibitor did not impair mast cell degranulation ( Supplementary Fig. 9 ). We next investigated whether contact with opsonized parasites could also trigger late activation events in hMCs such as cytokine and chemokine production. Opsonized parasites triggered hMCs to secrete CC-chemokine ligand 2 (CCL2), CCL4, CXC-chemokine ligand 8 (CXCL8), granulocyte-macrophage colony-stimulating factor (GM-CSF), TNF-α and interleukin (IL)-1β as measured by multiplex analysis of co-culture supernatants ( Fig. 7c ). Taken together, the above findings show that IgG-opsonized T. gondii induce mast cell ADDS resulting in tryptase-dependent parasite death and in hMC activation to cytokines and chemokine production. In the present work, we investigated the responses of hMCs to cell-bound antigens targeted by either IgE or IgG. We report that localized stimuli provided by cellular antigens trigger the polarized exocytosis of hMC granules at the cell–cell contact site resulting in a sustained exposure of granule-stored mediators at the synaptic contact. Remarkably, ADDS also occurs upon contact with IgG-opsonized T. gondii tachyzoites leading to tryptase-dependent parasite death and to the release of inflammatory cytokines and chemokines. For this study, we developed a method to monitor live mast cell degranulation using a combination of microscopy and flow cytometry approaches. In a first approach, we monitored mast cell degranulation following FcR aggregation using soluble anti-IgE. Time-lapse microscopy revealed that, although a fraction of exocyted granules was released in the extracellular milieu, a significant amount of granules stayed associated with the hMC surface independently of the strength of the applied stimulus. Moreover, measurement of degranulation at the cell population level showed that only a fraction of mast cells degranulated in response to FcR crosslinking (ranging from 30 to 70% of the cells in the different donors), in agreement with previously reported data [40] , [41] . The molecular mechanisms of functional heterogeneity of individual mast cells belonging to a phenotypically homogeneous population are presently elusive and are worth of further investigation. Previous data on mouse mast cells suggested that released granules might serve as vehicles to convey signals distantly from degranulated mast cells. It has been shown that heparin matrix protects mast cell mediators from degradation and influences tryptase and chymase bioactivities [8] , [13] . Moreover, Abraham and co-workers showed that the exocyted granules can serve as nanoparticles for progressive delivery of serglycin proteoglycans-embedded compounds such as TNF [11] , [12] . Conversely, an early study, based on biochemical approaches, reported that chymase and heparin are retained on the rat mast cell surface upon degranulation [10] . Our results extend previous data by showing the progressive accumulation of exocyted material on live hMC surface during the degranulation process. FACS analysis also showed that granule-stored chymase was detected on the mast cell surface for hours after degranulation, indicating that exposed granule matrix on hMC surface retained biological activity for sustained time. Our results thus reveal that hMCs themselves can serve as ‘bio-diffusers’ of stored mediators after degranulation. The observation that mast cells harbour on their surface degranulated biological material prompted us to investigate whether mast cells triggered by cell-bound antigens might dedicate their secretion to specific cellular partners. Our morphological approaches show that this is actually the case since following FcR triggering by cell-bound antigens a fraction of released granules remains on mast cell surface specifically in the area of cell–cell contact. This synaptic display of degranulated material might be instrumental to rapidly reach high concentration of bioactive mediators at the contact of targeted cell surface. The above results raise the question of how large amounts of diffusible mediators such as β-hexosaminidase might be released following synaptic contacts ( Fig. 2f ). We speculate that at high B-cell/mast cell ratios, several B cells might enter in contact with an individual mast cell simultaneously thus triggering a large fraction of FcεRI. Such a stimulation might be comparable to that induced by soluble anti-IgE. As β-hexosaminidase is not associated with the serglycin matrix [42] , it immediately diffuses in the extracellular medium independently of the stimulation condition. As a consequence, the amount of β-hexosaminidase measured in the cell supernatant is similar following both localized and non-polarized stimulation. As hMCs express two main activating FcR, FcεRI and FcγRIIA, we set-up experimental conditions to monitor triggering of each one of these receptors by cellular antigens. In either case, the local stimulation by cell-bound antigens induced a polarized degranulation restricted to the contact area between the two cells. To our knowledge, the mast cell activation by IgG-targeted cell-bound antigens we describe was not reported before. Unlike basophils, which express inhibitory FcγRIIB and therefore poorly respond to IgG immune complexes [43] , FcγRIIB expression is undetectable on hMC surface compatible with their efficient stimulation via IgG [24] . We studied in detail the polarized degranulation triggered via FcεRI crosslinking. We found that the local degranulation process was accompanied by a localized signalling area characterized by punctuated pTyr and pLAT staining. This observation is in line with previous studies in which FcεRI signalling was investigated using antigen displayed on supported lipid bilayers. Silverman et al . showed that FcεRI and the associated signalling components such as SLP76, Syk and LAT selectively cluster at the site of stimulation [31] . Carroll-Portillo et al . showed that FcR clusters are detectable at the mast cell/lipid bilayer contact area 1 min after stimulation and then, they coalesce leading to the formation of a mast cell synapse [32] . Using patterned lipid bilayers, Wu et al . reported that secretion is directed towards the substrate where the stimuli are located, but do not strictly co-localize with the signalling clusters [30] . In the present study, we employed techniques allowing visualize the exocyted material at the mast cell degranulatory synapse in live as well as in fixed conjugates. These methods have the advantage over classical immunofluorescence methods to provide a dynamic picture of the degranulation process during the sustained cell–cell interaction. When mast cells were stimulated by cell-bound antigens, fixed, permeabilized and stained for tryptase, we observed that only a small fraction of the total pool of mast cell granules was polarized ( Supplementary Fig. 10 ). These observations suggest that the synaptic mode of mast cell stimulation results in a local display of small amounts of granules over a prolonged time. In other words, when triggered by cell-bound ligands, mast cells appear to behave as lymphocytes that establish sustained productive synapses with target cells resulting in dedicated secretion. It is tempting to speculate that ADDS might, on one hand limit collateral damages to the microenvironment and on the other hand, dedicate mast cell secretion while sparing bioactive material. The dynamic picture of the degranulation process also allows to link the ongoing polarized exocytosis to FcR triggering. Our data extend data reported by Wu et al . who focused on localized endosomal recycling and not on mast cell degranulation [30] . In agreement with this and other reports [30] , [31] , [32] , we show that FcR and the associated signalling component LAT cluster in the proximity of the budding granules. These results, together with the observation of a localized clearance of actin cytoskeleton at the degranulatory synapse, provide a mechanistic link between localized signalling and polarized secretion. Accordingly, actin cytoskeleton disassembly was previously reported in rodent mast cells stimulated with soluble antigens [41] , [44] . This process was proposed to allow mast cell granules to cross the cortical actin ring and reach plasma membrane [45] . Mast cell degranulatory synapses present several differences when compared with the T-cell/ antigen-presenting cell (APC) immunological synapses. T-cell synapses are accompanied by T-cell MTOC and Golgi apparatus polarization towards the APC [46] . Moreover, both helper T cells and cytotoxic T cells are highly motile, both in vitro and in vivo , and reduce their locomotion when encountering cognate APC [47] , [48] . Mast cells exhibit a different behaviour. First, they undergo neither MTOC nor Golgi apparatus polarization towards the signalling area. The observation that polarized mast cell degranulation requires local signalling and cytoskeletal rearrangement rather than the whole re-polarization of the cell is in agreement with previous data showing that an extension of microtubules is sufficient to guide granules to plasma membrane [45] . Second, they are apparently poorly motile and form relatively loose synaptic contacts with antibody-targeted cells when compared with T-cell synapses [49] , [50] . Thus, differently from T cells that undergo a complete re-programming of their motility and polarization behaviour, mast cells release granules at the site of FcR triggering without profound changes in their motility. The fact that mast cells release a large number of secretory granules might contribute to create steric hindrance at the synaptic contact thus resulting in unstable, although sustained, contacts. These loose contacts might allow mast cell granules to escape the synaptic area (see Supplementary Movie 4 ) and allow the release of a substantial fraction of soluble bioactive compounds such as histamine and β-hexosaminidase ( Fig. 2 ). Mast cell activation by FcγR-triggering induced by cell-bound antigen has never been investigated. Nevertheless, this situation is very likely to happen in vivo . An interesting finding of our work is that FcγR-triggering by opsonized B cells or T. gondii tachyzoites results in degranulatory synapses. The fact that mast cells can be activated by interaction with IgG-targeted cells indicates that they might be specifically re-directed against pathogens, infected cells or cellular self-antigens in the course of in vivo immune responses. An example of mast cell capacity to respond to IgG-targeted pathogens comes from our results on T. gondii . Although mast cells incubated with non-opsonized tachyzoites did not show any sign of degranulation, in line with previous data [51] , opsonized tachyzoites induced a strong and polarized degranulation. Interestingly, exposure of parasite to mast cell granules upon synaptic contacts was accompanied by its death, which was at least partially dependent of a functional mast cell tryptase. This observation indicates that degranulatory synapses enable mast cell to display enough bioactive molecules at the contact with the parasite to elicit a cytotoxic effect. Involvement of soluble molecules is not excluded but contact with the parasite appears to be necessary to induce parasite death as T. gondii in contact with non-degranulated hMCs were still alive. Our results support the notion that mast cells might be effectors of the immune response against this intracellular pathogen and unveil a novel mechanism of mast cell control of parasite infection. Moreover, we show that when interacting with opsonized T. gondii mast cells release inflammatory cytokines and chemokines. As T. gondii infection results in cell death or impaired immune function [52] , we infer that the capacity to perform ADDS allows mast cells to defend themselves from tachyzoite infection and consequently to produce substantial amounts of inflammatory mediators. These mediators are expected to favour the recruitment and the activation of immune cells such as neutrophils and cytotoxic lymphocytes instrumental in the defence against the parasite. In summary, our results shed new light on mast cell biology by showing that in the presence of cellular antigens, both IgE and IgG can trigger synaptic activation of mast cells. The newly described capacity of mast cells to perform ADDS for dedicated secretion and defence reveals unpredicted functions of these cells that are worth of further investigation. Reagents Primary antibodies used for immunostaining (2 μg ml −1 ) were as follows: anti-FcγRIIA (clone IV.3, StemCell), anti-mast cell tryptase (clone G-12), anti-phosphotyrosine (clone PY99), anti-SAG-1 (clone TP3) all from Santa Cruz Biotechnology. Anti-α-tubulin (clone DM1A) was received from Sigma-Aldrich. Anti-GM130 (clone 35/GM130), anti-FcγRI (clone 10.1), anti-FcγRIII (clone 3G8), anti-CD117 (clone 104D2), anti-phospho-LAT (pY226) (clone J96-1238.58.93) all from BD Biosciences. Anti-mast cell chymase (clone B7) from Millipore and anti-FcεRI (clone AER-37) from eBioscience. Antibodies used to stimulate mast cell were as follows: human IgE (1 μg ml −1 , Abcam), anti-IgE (clone MH25-1, Santa Cruz) and humanized IgE anti-CD20 (1 μg ml −1 , InvivoGen). Humanized anti-CD20 IgG, Rituximab, from Roche. Alexa Fluor 488-labelled Phalloidin and all the secondary antibodies used (1 μg ml −1 , Alexa Fluor-conjugated) from Molecular Probes, Inc. In some experiments, cells were labelled with CellTrace Far Red DDAO-SE and CellTracker Blue CMAC (Molecular probes) according to the manufacturer’s instructions. Fixable Viability Dye efluor450 (Affymetrix, eBioscience) was used to irreversibly label dead cells prior fixation. Selective inhibitor of mast cell tryptase: APC 366 (Tocris Bioscience) and Chymase inhibitor: SBTI (Sigma) was used. Mast cell granule matrix was stained using avidin-sulforhodamine 101, avidin-FITC (Sigma) or avidin-Alexa488 (Invitrogen). Annexin-V-Alexa647 (Invitrogen) was used to monitor degranulation. Human mast cells Peripheral blood mononuclear cells were obtained from buffy coats (Etablissement Français du Sang). CD34 + precursors cells were isolated from peripheral blood mononuclear cells (EasySep Human CD34 Positive Selection Kit, STEMCELL Technologies). CD34 + cells were grown under serum-free conditions using StemSpan medium (STEMCELL Technologies) supplemented with recombinant human IL-6 (50 ng ml −1 ; Peprotech), human IL-3 (10 ng ml −1 ; Peprotech) and 3% supernatant of CHO transfectants secreting murine SCF (a gift from Dr P. Dubreuil, Marseille, France, 3% correspond to ~50 ng ml −1 SCF) for 1 week, we indeed previously showed that murine SCF can substitute human SCF for hMC generation [6] . Cells were grown in IMDM Glutamax I, sodium pyruvate, 2-mercaptoethanol, 0.5% BSA, Insulin-transferrin selenium (all from Invitrogen), ciprofloxacin (10 μg ml −1 ; Sigma-Aldrich), IL-6 (50 ng ml −1 ) and 3% supernatant of CHO transfectants secreting murine SCF for 8 weeks tested phenotypically (Tryptase + , CD117 + , FcεRI + ) and functionally (β-hexosaminidase release in response to FcεRI crosslinking) before use for experiments. Only primary cell lines showing more than 95% CD117 + /FcεRI + cells were used for experiments Cell opsonization Epstein–Barr virus-transformed lymphoblastoid cell line JY cells (ECACC No. : 94022533) were routinely passaged in RPMI 10% FCS. JY cells were opsonized with 1 μg ml −1 rituximab for 30 min at 37 °C as indicated. T. gondii tachyzoites (RH strain) were maintained by passage on confluent monolayers of human foreskin fibroblast. Tachyzoites were opsonized with 5 μg ml −1 IgG anti-SAG-1 for 30 min at 37 °C, washed and immediately used for experiments. Mast cell degranulation assays hMCs were sensitized or not with human IgE anti-CD20 (1 μg ml −1 ) for 16 h. The cells were then washed and distributed in 96-well flat-bottom plates at a density of 1 × 10 5 cells in 50 μl Tyrode’s buffer and adapted to 37 °C for 20 min. hMCs were then treated with either soluble goat anti-human IgE at indicated concentrations or different ratios of JY cells in 50 μl pre-warmed Tyrode’s buffer for 60 min at 37 °C, 5% CO 2 . Supernatants were harvested and β-hexosaminidase was assayed by measuring release of p-nitrophenol from the substrate p -nitrophenyl N -acetyl-β- D -glucosaminide as described [53] . The cells were next stained with 2.5 mmol l −1 avidin-FITC at 4 °C for 30 min then proceeded to flow cytometry analysis. For chymase exposure measurement, hMCs were previously sensitized with human IgE (1 μg ml −1 ) and stimulated with 2.5 μg ml −1 anti-IgE for 20 min. Cells were chilled at 4 °C and rested in culture medium at 37 °C for indicated times. Cells were stained for surface chymase expression and analysed on a FACSCalibur flow cytometer and FlowJo software (Tree Star, Inc.) was used to analyse the data. Confocal microscopy analysis of hMC degranulation A total of 5 × 10 4 hMCs previously sensitized with human IgE (1 μg ml −1 ) were plated on Poly- D -Lysine (Sigma)-coated Lab-Tek chambered coverglass (Nunc) in Tyrode’s buffer supplemented with 8 μg ml −1 avidin-sulforhodamine 101 (Av.SRho, highly cationic glycoprotein that selectively stains mast cell granules [34] ) or Annexin-V-Alexa647 (final 3% v/v) [35] as indicated and warmed at 37 °C for 20 min. Cells were stimulated with 2.5 μg ml −1 goat anti-human IgE at time=0. Fluorescence was acquired every 2.3 s using Zeiss LSM 710 confocal microscope and ZEN software, environmental chamber (37 °C and 5% CO2), × 63 Plan-Apochromat objective (1.4 oil). In other experiments, hMCs were stimulated as above onto Poly- D -Lysine-coated diagnostic slides (Thermo Scientific) for 30 min at 37 °C then fixed and stained for chymase and tryptase. The samples were mounted and examined using a Zeiss LSM 710 confocal microscope and ZEN software with a × 63 Plan-Apochromat objective (1.4 oil), electronic zoom 3. z-Stacks image were acquired with an interval of 0.4 μm. Time-lapse monitoring of B cell or tachyzoite/hMC interaction A total of 5 × 10 4 hMCs previously sensitized or not with human anti-CD20 IgE (1 μg ml −1 ) were plated on Poly- D -Lysine (Sigma)-coated Lab-Tek chambered coverglass (Nunc) in Tyrode’s buffer supplemented with 8 μg ml −1 avidin-sulforhodamine 101 (Av.SRho, highly cationic glycoprotein that selectively stains mast cell granules [34] , Sigma) or Annexin-V-Alexa647 (final 3% v/v) [35] as indicated and warmed at 37 °C for 20 min. According to experiments, either 5 × 10 4 DDAO-loaded JY cells or 5 × 10 4 DDAO-loaded and rituximab-opsonized JY cells or 1 × 10 6 opsonized or not tachyzoites were dropped onto 5 × 10 4 pre-warmed hMCs. Fluorescence was acquired every 2.3 s using Zeiss LSM 710 confocal microscope and ZEN software, environmental chamber (37 °C and 5% CO 2 ) and × 63 Plan-Apochromat objective (1.4 oil). Confocal microscopy analysis of JY cell/hMC conjugates A total of 2.5 × 10 4 hMCs sensitized or not with human anti-CD20 IgE (1 μg ml −1 ) were plated on Poly- D -Lysine-coated diagnostic slides (Thermo Scientific) in 25 μl Tyrode’s buffer supplemented with 8 μg ml −1 Av.SRho for 20 min at 37 °C. According to the experiments, either 2.5 × 10 4 JY cells or rituximab-opsonized JY cells (loaded with either DDAO or CellTracker Blue CMAC) were added and allowed to interact with hMCs for 30 min at 37 °C then fixed with 4% paraformaldehyde. Cells were permeabilized in PBS 1% BSA containing 0.1% saponin then stained for indicated molecules. The samples were mounted and examined using a Zeiss LSM 710 confocal microscope and ZEN software with a × 63 Plan-Apochromat objective (1.4 oil) and electronic zoom 3. Image quantification Scoring of the slides was performed in a blinded manner by evaluating for each condition at least 50 hMC/B-cell conjugates in randomly selected fields from at least three independent experiments. To evaluate the polarization of granules or GM130 towards the degranulatory synapse, unprocessed images were analysed using the Region Measurements function of the Metamorph software (Universal Imaging). Each hMC was divided into three equal regions by the software, one containing the degranulatory synapse (one-third of the hMC, region 1) and the other containing the two regions left (region 2, see schemes drawn on figures). To evaluate the polarization of granules towards T. gondii , the region 1 drawn represents the one-seventh of the cell containing the synaptic area. The software calculates the integrated fluorescence intensity in each region. For each conjugate, a ratio between the fluorescence in the synaptic region and the fluorescence in the whole cell (region 1/(region 1+region 2)) was calculated. To evaluate precisely the localization of FcεRI, pTyr pLAT and actin at the degranulatory synapse, two regions were analysed, one containing the degranulatory synapse (1/7 (for FcεRI, pTyr pLAT) or 1/20 (for actin) of the hMC, region 1, synaptic area) and the other containing the opposed region 2 (1/7 (for FcεRI, pTyr pLAT) or 1/20 (for actin) of the hMC, region 2, distal area, see schemes). The integrated fluorescence intensity calculated by the software in both regions are compared. Distances between MTOC and the centre of the synaptic area were measured using Zen software (see scheme). For three-dimensional quantification of the intensity of Av.SRho fluorescence, a series of z-stack of optical sections of hMC/B-cell conjugates were acquired. Av.SRho fluorescence was measured using the ROI statistics tool of the ICY software ( http://icy.bioimageanalysis.org ) on image projections in two equal defined volumes (see scheme in Supplementary Fig. 6 ). Analysis of T. gondii /hMCs conjugates For confocal microscopy, 5 × 10 4 hMCs were plated on Poly- D -Lysine-coated diagnostic slides (Thermo Scientific) in 25 μl Tyrode’s buffer supplemented with 16 μg ml −1 Av.A488 for 20 min at 37 °C. A total of 1 × 10 6 or 1 × 10 5 opsonized or not tachyzoites in 25 μl Tyrode’s buffer were co-cultured either for 1 h (hMC polarized degranulation analysis) or 4 h (tachyzoite cell death analysis) at 37 °C. For tachyzoites cell death analysis, hMCs were pretreated or not with tryptase (APC 366, 10 μmol l −1 ) or chymase (SBTI, 100 μg ml −1 ) inhibitors for 30 min. hMCs and tachyzoites were next co-cultured in Tyrode’s buffer supplemented or not with the same amount of inhibitors for 4 h. Cells were fixed with 4% paraformaldehyde then stained for SAG-1 antigen and with the fixable viability dye eFluor450 (eBiosciences). The samples were mounted and examined as above described. For flow cytometry analysis, 1 × 10 5 hMCs were co-cultured with 2 × 10 6 or 2 × 10 5 opsonized or not tachyzoites in 50 μl Tyrode’s buffer in 96-well U-bottomed plates for (i) 1 h at 37 °C then chilled at 4 °C and incubated with Av.A488 and Goat anti-mouse IgG2a-alexa 647 for SAG-1 staining or (ii) 4 h then chilled at 4 °C and stained for surface chymase exposure. Cells were analysed by FACScalibur as above described. Cytokine production measurement TNF-α, IL-1β, GM-CSF, CCL2 and CCL4 were measured by using CBA flex detection kits (BD-Pharmigen). CXCL8 was measured by sandwich ELISA (IL-8 ELISA Kit, Peprotech) according to the manufacturer’s instructions. Statistical analysis Unpaired or paired Student’s t -tests were used for comparing two groups (Prism 5, GraphPad Software). Data are expressed as means±s.e.m. ( P -value range is indicated: * P <0.05, ** P <0.01 and *** P <0.001). Flow cytometry profiles and microscopy images are representative of repeated experiments. How to cite this article : Joulia, R. et al . Mast cells form antibody-dependent degranulatory synapse for dedicated secretion and defence. Nat. Commun. 6:6174 doi: 10.1038/ncomms7174 (2015).